Proof of dual-topology architecture of Fluc F−channels with monobody blockers Fluc-type F − channels—used by microorganisms for resisting fluoride toxicity—are unusual in their quaternary architecture: they are thought to associate as dimers with the two subunits in antiparallel transmembrane orientation. Here, we subject this unusual structural feature to a direct test. Single purified Fluc channels recorded in planar lipid bilayers are constitutively open, with rare, short-lived closings. Using combinatorial libraries, we generated synthetic binding proteins, ‘monobodies,’ that specifically bind to Fluc homologues with nanomolar affinity. Reversible binding of monobodies to two different Fluc channel homologues is seen in single-channel recordings as long-lived nonconducting events that follow bimolecular kinetics. By applying monobodies sequentially to the two sides of the bilayer in a double-sided perfusion manoeuvre, we show that Fluc channels present monobody-binding epitopes to both sides of the membrane. The result establishes that Fluc subunits are arranged in dimeric antiparallel orientation. Ion channels of the newly discovered Fluc family [1] , [2] protect unicellular microorganisms against the toxicity of aqueous F − anion, an environmentally ubiquitous inhibitor of key enzymes in energy production and nucleic acid synthesis [3] . These F − -specific channels keep cytoplasmic F − below inhibitory levels by undermining the weak-acid accumulation effect of hydrofluoric acid that would otherwise occur in acidic niches encountered by bacteria, yeasts and protozoa [2] , [4] , [5] . Fluc channels function as dimers of small polypeptides (~130 residues) containing four transmembrane segments each, and mutually reinforcing lines of indirect evidence suggest that the two subunits are arranged in an antiparallel transmembrane orientation [2] . Though unprecedented among ion channels, dual-topology dimeric architecture is known in the multidrug efflux pump EmrE [6] , [7] , [8] , [9] , and many membrane transport proteins adopt an analogous motif, the inverted structural repeat, within a single polypeptide chain [10] . We were therefore motivated to determine the quaternary architecture of Fluc channels unambiguously. The many years of controversy [11] over parallel versus antiparallel assembly of EmrE highlight the difficulties of distinguishing these alternative architectures. Engineered binding proteins have proven powerful in mechanistic and structural investigations of membrane proteins [12] , [13] . By combining single-channel recording with specific Fluc channel blockers selected from combinatorial libraries by protein engineering technologies, we now unequivocally establish the antiparallel arrangement of Fluc channels functioning in phospholipid membranes. Selection of Fluc-directed monobodies In ongoing efforts to develop crystallization chaperones suitable for structure determination, we generated engineered binding proteins termed ‘monobodies’ for two bacterial Fluc homologues, named Ec2 and Bpe [2] . Monobodies are single-domain proteins of ~10 kDa, derived from the tenth fibronectin type III domain of human fibronectin [14] , [15] . They are selected from two different combinatorial phage-display libraries ( Fig. 1a ), termed ‘loop’ and ‘side,’ in which 16–26 positions are diversified using highly tailored amino acid compositions followed by gene shuffling and further selection in the yeast-display format [16] . These water-soluble, stably folded, cysteine-free, β-sheet proteins bind specifically to their targets with submicromolar dissociation constants. 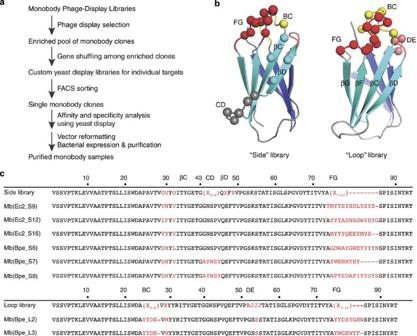Figure 1: Selection of Fluc-directed monobodies. (a) Outline of monobody selection strategy. (b) Structure of monobody scaffold, showing residues (spheres) varied in combinatorial side and loop libraries. (c) Sequences of monobodies (variable regions in red) selected against Fluc homologues Ec2 and Bpe from side and loop libraries as indicated by ‘S’ or ‘L’ designators in monobody labels. All eight monobodies bind to their targets with submicromolar dissociation constants, and all except Mb(Bpe_S8) block Fluc channels in electrical recording assays. Upper sequence of each library indicates tailored variation as follows: ‘X’ denotes a mixture of 30% Tyr, 15% Ser, 10% Gly, 5% Phe, 5% Trp and 2.5% each of all the other amino acids except for Cys; ‘B’, a mixture of Gly, Ser and Tyr; ‘J’, a mixture of Ser and Tyr; ‘O’, a mixture of Asn, Asp, His, Ile, Leu, Phe, Tyr and Val; ‘U’, a mixture of His, Leu, Phe and Tyr; ‘Z’, a mixture of Ala, Glu, Lys and Thr, as previously reported16. Figure 1 shows sequences of the monobodies selected against each homologue, as well as the locations of the loop and side residue variations on the protein surface. Figure 1: Selection of Fluc-directed monobodies. ( a ) Outline of monobody selection strategy. ( b ) Structure of monobody scaffold, showing residues (spheres) varied in combinatorial side and loop libraries. ( c ) Sequences of monobodies (variable regions in red) selected against Fluc homologues Ec2 and Bpe from side and loop libraries as indicated by ‘S’ or ‘L’ designators in monobody labels. All eight monobodies bind to their targets with submicromolar dissociation constants, and all except Mb(Bpe_S8) block Fluc channels in electrical recording assays. Upper sequence of each library indicates tailored variation as follows: ‘X’ denotes a mixture of 30% Tyr, 15% Ser, 10% Gly, 5% Phe, 5% Trp and 2.5% each of all the other amino acids except for Cys; ‘B’, a mixture of Gly, Ser and Tyr; ‘J’, a mixture of Ser and Tyr; ‘O’, a mixture of Asn, Asp, His, Ile, Leu, Phe, Tyr and Val; ‘U’, a mixture of His, Leu, Phe and Tyr; ‘Z’, a mixture of Ala, Glu, Lys and Thr, as previously reported [16] . Full size image Monobodies block Fluc channels A small molecular size, short loops between transmembrane segments and stubby hydrophilic termini conspire to limit the amount of surface that Fluc channels can expose to aqueous solution. This limitation anticipates that in some cases a monobody’s footprint on the channel might lie close to the pore entryway or might even cover it. We were not entirely surprised, therefore, to find that seven of the eight monobodies used for crystallization trials also inhibit F − current through the Fluc homologues against which they were selected. This effect is illustrated for both homologues under study here, with two different monobodies for each, in single-channel recordings in planar phospholipid bilayers ( Fig. 2 ). Whereas Fluc channels are nearly always open under our recording conditions [2] , the monobodies at submicromolar concentrations produce stochastic nonconducting ‘block’ events in the seconds-to-minutes range, kinetic details varying with the particular monobody tested. These recordings also attest to the specificity of the monobodies, since Bpe-directed monobodies at high concentration exert no effect on Ec2, and vice versa. To our knowledge, these monobodies are the highest-affinity specific inhibitors of any known anion channel. 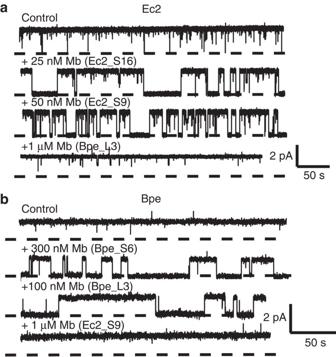Figure 2: Specific block of Fluc channels by monobodies. Fluc homologues Ec2 (a) or Bpe (b) were inserted into planar lipid bilayers for single-channel recording at −200 mV in the presence of indicated monobody, using low protein density liposomes (0.05 μg Fluc per mg lipid). Dashed lines represent zero current, and openings are shown upward. Figure 2: Specific block of Fluc channels by monobodies. Fluc homologues Ec2 ( a ) or Bpe ( b ) were inserted into planar lipid bilayers for single-channel recording at −200 mV in the presence of indicated monobody, using low protein density liposomes (0.05 μg Fluc per mg lipid). Dashed lines represent zero current, and openings are shown upward. Full size image We chose one of the channel-monobody pairs, Bpe//Mb(Bpe_L3), for a quantitative examination of the blocking process. Single-channel recordings ( Fig. 3a ) in the presence of this monobody (henceforth abbreviated ‘L3’) show that both blocked and open intervals are exponentially distributed ( Fig. 3b ), with time constants τ B and τ o , respectively. Open times shorten and block times remain constant as monobody concentration increases ( Fig. 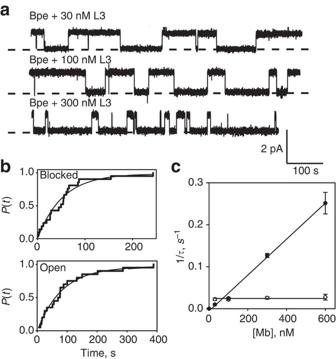Figure 3: Bimolecular kinetics of monobody block. (a) Single Bpe recordings with indicated concentrations of monobody L3 incischamber, with conditions as inFig. 2. (b) Cumulative distributions of blocked and open dwell times (n=20 for each) for a single Bpe channel in the presence of 30 nM L3 monobody. Solid lines show single-exponential fits. (c) Dependence of blocked (open points) and open (closed points) time constants on monobody concentration [Mb], for L3 block of Bpe. Each point represents mean ± s.e.m. time constant from three to six separate bilayers. Solid lines show fits to equation (1a) and equation (1b) for open and blocked intervals, respectively, withτB=41 s (koff=0.025 s−1),τO=77 s (kon=4.3 × 105s−1M−1),KD=58 nM. 3c ), in quantitative agreement with expectations of a bimolecular blocking scheme with rate constants of blocker association ( k on ) and dissociation ( k off ): Figure 3: Bimolecular kinetics of monobody block. ( a ) Single Bpe recordings with indicated concentrations of monobody L3 in cis chamber, with conditions as in Fig. 2 . ( b ) Cumulative distributions of blocked and open dwell times ( n =20 for each) for a single Bpe channel in the presence of 30 nM L3 monobody. Solid lines show single-exponential fits. ( c ) Dependence of blocked (open points) and open (closed points) time constants on monobody concentration [Mb], for L3 block of Bpe. Each point represents mean ± s.e.m. time constant from three to six separate bilayers. Solid lines show fits to equation (1a) and equation (1b) for open and blocked intervals, respectively, with τ B =41 s ( k off =0.025 s −1 ), τ O =77 s ( k on =4.3 × 10 5 s −1 M −1 ), K D =58 nM. Full size image Kinetic parameters and corresponding equilibrium dissociation constant are reported in the legend of Fig. 3 . Channel block may reflect physical pore occlusion by the monobody, but evidence for this is weakly suggestive at best; the results do not rule out an allosteric inhibition mechanism. Sidedness of monobody block We consistently observe single-channel block regardless of the side of the bilayer to which monobody is added. This finding would be perplexing if the channel were constructed with its two subunits in parallel transmembrane assembly, since in the liposomes used for fusion into planar bilayers, roughly half of the Fluc amino termini are exposed to the liposome interior and half to the outside solution [2] . In contrast, the observation is in natural harmony with antiparallel assembly, wherein the monobody-binding surface on the dimeric channel—its epitope—would be exposed twice, once to each side of the membrane ( Fig. 4a ). 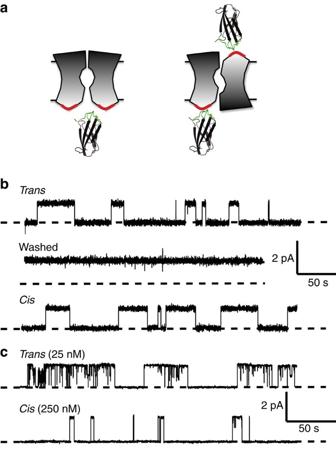Figure 4: Two-sided exposure of monobody epitope. (a) Cartoon contrasting the presentation of monobody-binding epitopes (red surface) in channels with parallel or antiparallel architecture. (b) Sequential recordings of the same single Bpe channel with 100 nM monobody L3 initially on thetransside at 200 mV (upper trace), after washingtransmonobody away (middle trace), and, after switching holding voltage to −200 mV, with 100 nM monobody L3 subsequently added to thecisside (lower trace). Dissociation constants estimated from limited records such as these were: 70 and 110 nM forcis- andtrans-addition, respectively. (c) Analogous experiment with single Ec2 channel in the presence of 25 nM Mb(Ec2_S9) on thetransside (upper trace). After extensivetrans-side perfusion to remove the monobody, the monobody was added to thecischamber at 10-fold higher concentration (lower trace). Figure 4: Two-sided exposure of monobody epitope. ( a ) Cartoon contrasting the presentation of monobody-binding epitopes (red surface) in channels with parallel or antiparallel architecture. ( b ) Sequential recordings of the same single Bpe channel with 100 nM monobody L3 initially on the trans side at 200 mV (upper trace), after washing trans monobody away (middle trace), and, after switching holding voltage to −200 mV, with 100 nM monobody L3 subsequently added to the cis side (lower trace). Dissociation constants estimated from limited records such as these were: 70 and 110 nM for cis - and trans -addition, respectively. ( c ) Analogous experiment with single Ec2 channel in the presence of 25 nM Mb(Ec2_S9) on the trans side (upper trace). After extensive trans -side perfusion to remove the monobody, the monobody was added to the cis chamber at 10-fold higher concentration (lower trace). Full size image To definitively ascertain the sidedness of epitope exposure, we performed two-sided perfusion experiments on single Bpe channels ( Fig. 4b ). Channel block was recorded in the presence of monobody L3 added to one side of the membrane (upper trace). The blocker was then washed away by extensive perfusion, as confirmed by the subsequent absence of blocking events (middle trace). Finally, with the same channel molecule in the bilayer, monobody was added to the opposite side of the membrane. Blocking events of similar duration were again observed (lower trace), a result demonstrating that the channel’s epitope appears on both sides of the membrane. In these experiments, we took care to switch the holding voltage polarity along with the side of monobody addition to insure that the blocker would ‘see’ the same voltage regardless of its side of action. Repeats of this experiment and minor variations thereof with either Fluc homologue always produce the same result: monobody-induced blocking events from both sides of the membrane, as additionally illustrated for block of Ec2 ( Fig. 4c ). The use of single channels here is particularly powerful in establishing Fluc antiparallel architecture, but it is nevertheless worthwhile to test a prediction of this picture: that monobody at high concentration should block macroscopic currents fully, regardless of the side to which it is added. This expectation is confirmed ( Fig. 5 ). Macroscopic Fluc current was recorded in bilayers containing hundreds or thousands of Bpe channels, and in all bilayers tested, monobody L3 added into the upper, cis , chamber of the bilayer system inhibits along a single-site curve approaching complete block at high concentration; the monobody added on the opposite trans side also produces full inhibition over the same concentration range. 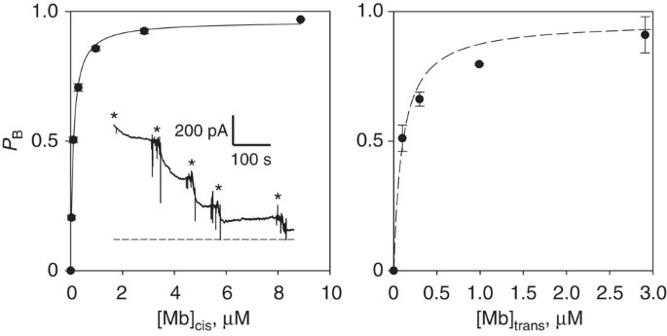Figure 5: Monobody block of macroscopic Fluc-Bpe current. Liposomes reconstituted with a high density of Fluc protein (10 μg Bpe per mg lipid) were fused into planar lipid bilayers. Current was allowed to stabilize, typically between 500 pA and 4 nA, before addition of monobody L3 to the chamber. Each point (mean±s.e.m.) represents fractional block of initial current in three to five separate bilayers. Left panel: addition to thecischamber, with single-site inhibition curve withKD=100 nM and maximal block=0.96. Inset: representative macroscopic titration recording with successive additions of L3 to total concentrations of 30 nM, 100 nM, 300 nM, 1 μM and 3 μM indicated by the asterisks; zero-current level marked by the dashed line. Right panel: addition to thetranschamber, with the samecis-inhibition function shown as dashed curve. Figure 5: Monobody block of macroscopic Fluc-Bpe current. Liposomes reconstituted with a high density of Fluc protein (10 μg Bpe per mg lipid) were fused into planar lipid bilayers. Current was allowed to stabilize, typically between 500 pA and 4 nA, before addition of monobody L3 to the chamber. Each point (mean±s.e.m.) represents fractional block of initial current in three to five separate bilayers. Left panel: addition to the cis chamber, with single-site inhibition curve with K D =100 nM and maximal block=0.96. Inset: representative macroscopic titration recording with successive additions of L3 to total concentrations of 30 nM, 100 nM, 300 nM, 1 μM and 3 μM indicated by the asterisks; zero-current level marked by the dashed line. Right panel: addition to the trans chamber, with the same cis -inhibition function shown as dashed curve. Full size image Discussion These double-sided channel-blocking experiments demonstrate that homodimeric Fluc channels present their monobody-binding epitopes to both sides of the membrane simultaneously. This fact is inconsistent with the parallel-subunit assembly by which nearly all ion channel proteins are constructed, but it is expected of antiparallel architecture. Indeed, the result is actually demanded for a symmetric antiparallel homodimer, wherein the subunits adopt identical conformations. However, our results do not rule out an asymmetric antiparallel homodimer, as in EmrE [6] , [8] , [9] , a point that will require extensive future analysis of two-sided channel block. Skeptics might object that these experiments fail to disprove parallel architecture because the epitope surfaces exposed to the two sides of the bilayer could arise from different channel sequences. We consider such a possibility plainly untenable, given the extreme rarity of obtaining Fluc-binding monobodies—on the order of 10 blockers selected from 10 billion variants—and from their high affinity and specificity of block, as indicated by the lack of monobody cross-reactivity between our two Fluc homologues. Several basic questions regarding details of monobody action remain unaddressed here. For instance, we have no information on whether the two epitopes on opposite sides of the Fluc channel can be simultaneously occupied by monobodies. Likewise, the mechanism of monobody block—physical pore-plugging or allosteric pore-closure—is unknown. While these intriguing biophysical issues will require detailed future examination, they have no bearing on our inferences about Fluc’s unusual quaternary architecture; the mechanistic minutiae of monobody block stand entirely apart from the design of and structural conclusions from the experiments presented here. Biochemical procedures and single-channel recording We used two bacterial Fluc channel homologues, nicknamed Ec2 and Bpe (sequences 35% identical, 68% similar), whose molecular characteristics, expression, purification and reconstitution into liposomes and planar lipid bilayers were recently described in detail [2] . The Ec2 construct is the wild-type sequence, while the Bpe construct carries two mutations, R29K and E94S, which improve biochemical tractability but do not alter the channel’s functional characteristics. Hexahistidine tags were removed from Bpe preparations by a 2-h treatment with lysine endoproteinase C (0.1 U mg −1 Bpe). All single-channel recordings used symmetrical solutions containing 300 mM NaF, 15 mM Mops-NaOH, 50 μg ml −1 bovine serum albumin, pH 7.0, in a horizontal planar bilayer chamber allowing two-sided perfusion [17] . Reconstituted proteoliposomes were produced by detergent dialysis at Fluc protein density of 0.05 or 10 μg mg −1 lipid for single-channel or many-channel experiments, respectively. Channels were fused into the bilayers by dropping ~0.5 μl of a proteoliposome suspension onto the upper, ‘ cis ’ side of the planar bilayer, with the opposite ‘ trans ’ chamber defined as electrical ground. Monobodies were stirred into the cis chamber or perfused into the trans chamber, and were removed from either chamber by extensive perfusion. Recordings were sampled at 2 kHz and bessel-filtered at 500 Hz, and monobody-blocking records were analysed in Clampfit 9 software after heavier digital filtering (50–100 Hz) to remove rare millisecond-timescale spontaneous closing events. By our display convention, all single-channel recordings are shown with opening upward, regardless of the voltage polarity. Blocking and dissociation rate constants were determined from dwell-time distributions of open and blocked intervals, respectively. Because block times are long-lived, on the order of a minute, only a small number of events could be logged in a given single-channel experiment. Accordingly, at least 20 events were always collected in a run, sufficient to obtain time constants from single-exponential fits to the cumulative dwell-time distributions. Rate constants were calculated from such time constants determined in three to six independent runs in separate bilayers. Monobody generation General methods for phage- and yeast-display library sorting and gene shuffling have been described [15] , [16] . The His-tagged Fluc homologues solubilized in detergent were mixed with an equimolar concentration of BTtrisNTA, a high-affinity His-tag ligand conjugated with biotin [18] , so as to capture the target proteins with streptavidin magnetic beads in phage-display selection and to detect them with fluorescent dye-labelled streptavidin in yeast surface display experiments [15] , [16] . Two separate monobody libraries, denoted ‘loop’ and ‘side,’ were used to generate monobodies with diverse binding-surface topography [16] . Four rounds of phage-display library sorting were performed using the target concentrations of 100, 100, 50 and 50 nM, for the first, second, third and fourth rounds in 100 mM NaCl, 10 mM NaF, 5 mM decylmaltoside, 25 mM Hepes-NaOH pH 7 at room temperature. A single round of yeast-display library sorting using a fluorescence-activated cell sorter (FACSAria, BD) was performed with 50 nM Fluc homologue. Affinity measurements were performed by titrating target protein//BTtrisNTA complexes in the yeast-display format in the above solution supplemented with 1 mg ml −1 bovine serum albumin at 4 °C as described previously [15] , [16] . Monobody proteins were expressed in E . coli using expression vector pHFT2 (ref. 19) [19] , and while bound to Talon beads, amino-terminal His tags were removed by a 16-h treatment with TEV protease (0.1 mg per 10 mg monobody). The eluate was concentrated and protein purified on Superdex-75 size exclusion columns. How to cite this article: Stockbridge, R. B. et al. Proof of dual-topology architecture of Fluc F − channels with monobody blockers. Nat. Commun. 5:5120 doi: 10.1038/ncomms6120 (2014).